Aldara activates TLR7-independent immune defence Aldara is a cream used for topical treatment of non-melanoma skin cancer, and is thought to act through stimulation of anti-tumour immunity. The active ingredient, imiquimod, has been shown to stimulate toll-like receptor 7. Aldara also induces psoriasis-like lesions when applied to naive murine skin, and as such is used as a mouse model for psoriasis. Here we find that in naive murine skin, Aldara induces inflammation largely independently of toll-like receptor 7. Surprisingly, inflammasome activation, keratinocyte death and interleukin 1 release also occur in response to the vehicle cream in the absence of imiquimod. We show that isostearic acid, a major component of the vehicle, promotes inflammasome activation in cultured keratinocytes, and so may contribute to the observed effects of Aldara on murine skin. Aldara therefore stimulates at least two immune pathways independently, and both imiquimod and vehicle are required for a full inflammatory response. Although it remains to be tested, it is possible that imiquimod-independent effects also contribute to the therapeutic efficacy of Aldara. Topical treatment with Aldara, a pharmaceutical preparation of cream containing 5% of the toll-like receptor 7 (TLR7)-agonist imiquimod (IMQ), results in tumour regression in up to 90% of patients with non-melanoma skin cancer (NMSC), that is, superficial basal cell carcinoma (BCC) or the precursor lesion actinic keratosis (AK) [1] , [2] , [3] . Observations in BCC and AK patients suggest that recruitment of plasmacytoid dendritic cells (pDCs) into the malignant tissue is responsible for the therapeutic effect [4] , [5] , [6] . Recently, it was shown that Aldara treatment resulted in pDC-mediated tumour killing in a murine melanoma model [7] . We and others previously showed that treatment with IMQ and Aldara resulted in upregulation of MHC class I on tumour cells, recruitment of T cells into the tumour, enhancement of their effector function and mobilization of Langerhans cells and inflammatory DCs, as well as in interleukin (IL)-17 production by dermal γδ-T cells [8] , [9] , [10] , [11] , [12] . In addition to effects on immune cells, direct pro-apoptotic effects of Aldara/IMQ on tumour cells have been described [5] , [13] , [14] , [15] . Because keratinocytes do not express TLR7 [7] , [16] , [17] , they presumably cannot respond directly to IMQ. Nevertheless, effects on keratinocytes have been described, such as induction of the secretion of IL-6, IL-8, TNFα and IL-1β by human primary keratinocytes in vitro , most likely via signalling through adenosine receptors [15] , [18] , [19] . Psoriasis-like lesions occur in susceptible patients with NMSC as a side effect of Aldara therapy [20] , [21] . Currently, repeated topical application of Aldara is considered a valuable mouse model for psoriasis [22] , which is an inflammatory and hyperproliferative condition of the skin. In psoriasis patients as well as in Aldara-treated mice, pDCs and neutrophils have been demonstrated to infiltrate the lesion site, and the cytokines IL-17, IL-22 and IL-23, as well as the presence of γδ-T cells, are considered as being important [8] , [23] , [24] , [25] . We set out to dissect the initial and local events in mice and NMSC patients following topical application of Aldara, to better understand the therapeutic mode of action in NMSC, as well as the events that mediate psoriasis-like lesions. Surprisingly, we found that Aldara induces a plethora of inflammatory reactions that are independent of TLR7 and even of its active component IMQ. Our results raise the possibility that the therapeutic effects of Aldara in NMSC may also be a result of both IMQ-dependent and IMQ-independent responses. Aldara causes TLR7-independent acanthosis Topical application of Aldara, a cream containing 5% of the TLR7-agonist IMQ, is an effective treatment for BCC and AK, and its major mode of action is thought to be TLR7 dependent. Indeed, topical application of Aldara results in increased infiltration of pDCs, a cell type that expresses high levels of TLR7 and is the main producer of type I interferon (IFN) [6] . Furthermore, Aldara induces local psoriasis-like symptoms in susceptible humans and in mice, such as inflammation, thickening and scaling of the skin [20] , [21] , [22] . To determine whether these depend on TLR7 and type I IFN, we topically treated shaved back skin of naive WT129, A129, C57BL/6 and TLR7-knockout (ko) mice with Aldara and analysed epidermal thickness, keratinocyte proliferation and differentiation. Using histomorphometry, we observed progressive acanthosis (epidermal thickening) starting 24 h after the first application of Aldara that was independent of type I IFN and TLR7 ( Fig. 1 ). Furthermore, Ki67 staining revealed hyperproliferation of basal keratinocytes 24 h after one topical Aldara application. Proliferation of suprabasal keratinocytes, which are normally quiescent, was also seen after Aldara treatment, in particular after 1 week ( Fig. 1b ). Twenty-four hours after one Aldara treatment, mice showed signs of parakeratosis, a differentiation abnormality of the interfollicular epidermis characterized by the presence of nucleated keratinocytes in the stratum corneum . Parakeratosis was independent of type I IFN and TLR7, but was influenced by the genetic background, because it was more pronounced in WT129 and A129 than in C57BL/6 and TLR7-ko mice after 1 week of treatment ( Fig. 1 ). In agreement with this, we observed significant alterations in keratinocyte differentiation ( Supplementary Fig. S1 ). Twenty-four hours after one Aldara treatment, expression of keratin 10 (K10), K14 and loricrin appeared to be normal; at later time points, however, they were more broadly distributed, and especially K14 appeared weaker, but was expressed in the entire epidermis and was no longer restricted to the basal layer. In addition, K10 and loricrin were strongly expressed in the hair follicles at day 7, whereas K6 and K16 were no longer restricted to the hair follicles, but were also expressed in the interfollicular epidermis ( Supplementary Fig. S1 ). This abnormal expression pattern is a hallmark of hyperproliferative conditions as seen in psoriasis [26] . 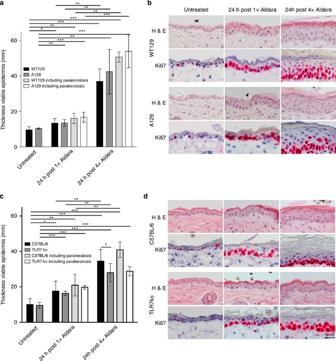Figure 1: Aldara induces type I IFN- and TLR7-independent keratinocyte acanthosis and hyperproliferation. (a,c) Quantification of acanthosis in the epidermis of WT129, A129, C57BL/6 and TLR7-ko mice. Error bars indicate s.d.; *P<0.05, **P<0.01 and ***P<0.001 (unpaired Student’st-test),n=5, 2 separate experiments. (b,d) Hematoxylin and eosin (H&E) and Ki67 staining of skin of untreated or Aldara-treated WT129, A129, C57BL/6 and TLR7-ko mice. Scale bar, 50 μm. Figure 1: Aldara induces type I IFN- and TLR7-independent keratinocyte acanthosis and hyperproliferation. ( a , c ) Quantification of acanthosis in the epidermis of WT129, A129, C57BL/6 and TLR7-ko mice. Error bars indicate s.d. ; * P <0.05, ** P <0.01 and *** P <0.001 (unpaired Student’s t -test), n =5, 2 separate experiments. ( b , d ) Hematoxylin and eosin (H&E) and Ki67 staining of skin of untreated or Aldara-treated WT129, A129, C57BL/6 and TLR7-ko mice. Scale bar, 50 μm. Full size image Although these results clearly demonstrate that the local effects of Aldara are independent of type I IFN and TLR7, topical treatment with Aldara resulted in rapid mobilization of pDC and high levels of type I IFN in the blood and ultimately in splenomegaly [22] ( Supplementary Figs S2 and S3 ). We showed that these systemic effects were dependent on TLR7 and type I IFN ( Supplementary Figs S2 and S3 ). Increased IFNα levels and pDC mobilization were transient as this response decreased already after the second treatment and was not measurable anymore after the third treatment. The transient nature of this response maybe because of exhaustion of common myeloid precursors (c-kit + , sca-1 − and lin − ) in the bone marrow of Aldara-treated mice, starting 6 h after one application ( Supplementary Fig. S4 ). In addition, it was recently shown that type I IFN negatively controls pDC numbers [27] . Keratinocyte proliferation upon Aldara-induced apoptosis To investigate how Aldara induces proliferation of basal keratinocytes as rapidly as 24 h after one topical application, and whether the release of cytokines by dying keratinocytes was a mediating factor, we performed transmission electron microscopy 12 h and 24 h after one Aldara treatment of murine skin. Starting at 12 h, Aldara massively disturbed the epidermal integrity and led to keratinocyte apoptosis as demonstrated by the presence of pyknosis, nuclear fragmentation and residual bodies ( Fig. 2a ). As the organelles such as mitochondria were intact in dying keratinocytes and we hardly observed cytolysis, we exclude necrosis as a mechanism of cell death. Notably, apoptosis did not occur specifically in keratinocytes but we also observed apoptotic Langerhans cells and degenerated axon endings ( Supplementary Fig. S5 ). 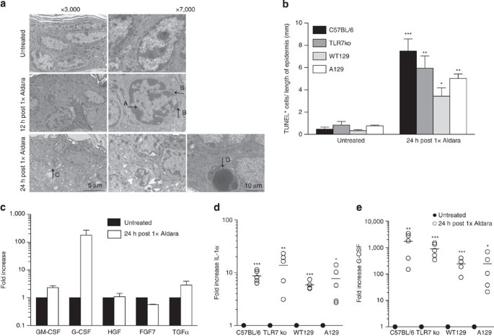Figure 2: Aldara induces apoptosis and cytokine upregulation. (a) Transmission electron microscopy of untreated skin of WT129 mice, and 12 h and 24 h after one topical Aldara application, respectively. The arrows indicate: (A) early-stage apoptotic pyknotic constricted nucleus, (B) intact mitochondria, (C) late-stage apoptotic pyknotic constricted nucleus and (D) residual body. Scale bar, 5 μm for × 3000 magnifications and 10 μm for × 7000 magnifications, respectively. (b) Quantification of epidermal TUNEL-positive cells 24 h after one topical Aldara application of the indicated mouse strains. Data are derived from following experimental groups: untreated C57BL/6 and TLR7-kon=4, WT129n=3, A129,n=2; treated C57BL/6, TLR7-ko, WT129n=5, A129n=4, and from 2–3 independent experiments, statistical significance displayed for counts of Aldara-treated samples compared with untreated samples of the same strain; error bars represent s.d. Display of fold increases in mRNA expression levels of various keratinocyte mitogens in Aldara-treated skin compared with untreated skin of levels of various keratinocytes mitogens (c),Il-1α(d) andG-csf(e) in the skin of WT129, A129, C57BL/6 and TLR7-ko mice (d,e) and C57BL/6 (c) assessed by qPCR 24 h after one topical Aldara treatment.n>4, 2–3 independent experiments, statistical significance displayed for ΔCT values of Aldara-treated compared with untreated samples of the same strain; *P<0.05, **P<0.01 and ***P<0.001 (unpaired Student’st-test). FGF7, fibroblast growth factor 7; GM-CSF, granulocyte-macrophage colony-stimulating factor; HGF, hepatocyte growth factor; TGFα, transforming growth factor α. Figure 2: Aldara induces apoptosis and cytokine upregulation. ( a ) Transmission electron microscopy of untreated skin of WT129 mice, and 12 h and 24 h after one topical Aldara application, respectively. The arrows indicate: (A) early-stage apoptotic pyknotic constricted nucleus, (B) intact mitochondria, (C) late-stage apoptotic pyknotic constricted nucleus and (D) residual body. Scale bar, 5 μm for × 3000 magnifications and 10 μm for × 7000 magnifications, respectively. ( b ) Quantification of epidermal TUNEL-positive cells 24 h after one topical Aldara application of the indicated mouse strains. Data are derived from following experimental groups: untreated C57BL/6 and TLR7-ko n =4, WT129 n =3, A129, n =2; treated C57BL/6, TLR7-ko, WT129 n =5, A129 n =4, and from 2–3 independent experiments, statistical significance displayed for counts of Aldara-treated samples compared with untreated samples of the same strain; error bars represent s.d. Display of fold increases in mRNA expression levels of various keratinocyte mitogens in Aldara-treated skin compared with untreated skin of levels of various keratinocytes mitogens ( c ), Il-1α ( d ) and G-csf ( e ) in the skin of WT129, A129, C57BL/6 and TLR7-ko mice ( d , e ) and C57BL/6 ( c ) assessed by qPCR 24 h after one topical Aldara treatment. n >4, 2–3 independent experiments, statistical significance displayed for ΔCT values of Aldara-treated compared with untreated samples of the same strain; * P <0.05, ** P <0.01 and *** P <0.001 (unpaired Student’s t -test). FGF7, fibroblast growth factor 7; GM-CSF, granulocyte-macrophage colony-stimulating factor; HGF, hepatocyte growth factor; TGFα, transforming growth factor α. Full size image In addition, we observed localized areas of apoptotic keratinocytes by TdT-mediated dUTP nick end labeling (TUNEL) staining at 24 h in all mouse strains ( Fig. 3a ). Quantification of TUNEL-stained cells in the non-lesional epidermis showed that Aldara-induced cell death was largely independent of type I IFN and TLR7 signalling ( Fig. 2b ). 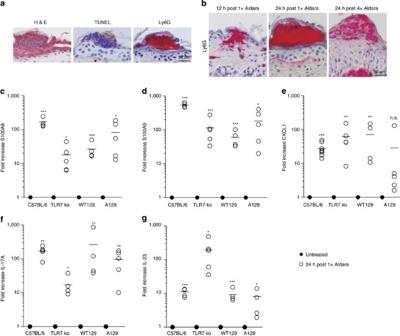Figure 3: Aldara induces abscess-like structures and neutrophil recruitment. (a) Representative staining of abscess-like structures with apoptotic cells in the epidermis of WT129 mice; Hematoxylin and eosin (H&E) (left), TUNEL (middle) and Ly6G (right), 24 h after 1 × Aldara. Scale bar, 50 μm. (b) Representative images of Ly6G staining at various time points after Aldara treatment of WT129 mice. Scale bar, 50 μm. Display of fold increases in mRNA expression levels of Aldara-treated skin compared with untreated skin ofS100A8(c),S100A9(d),Cxcl1(e),Il-17A(f) andIl-23(g) in the skin of WT129, A129, C57BL/6 and TLR7-ko, assessed by qPCR 24 h after one topical Aldara treatment. Statistical significance displayed for ΔCT values of Aldara-treated compared with untreated samples of the same strain; *P<0.05, **P<0.01, ***P<0.001 (unpaired Student’st-test). Figure 3: Aldara induces abscess-like structures and neutrophil recruitment. ( a ) Representative staining of abscess-like structures with apoptotic cells in the epidermis of WT129 mice; Hematoxylin and eosin (H&E) (left), TUNEL (middle) and Ly6G (right), 24 h after 1 × Aldara. Scale bar, 50 μm. ( b ) Representative images of Ly6G staining at various time points after Aldara treatment of WT129 mice. Scale bar, 50 μm. Display of fold increases in mRNA expression levels of Aldara-treated skin compared with untreated skin of S100A8 ( c ), S100A9 ( d ), Cxcl1 ( e ), Il-17A ( f ) and Il-23 ( g ) in the skin of WT129, A129, C57BL/6 and TLR7-ko, assessed by qPCR 24 h after one topical Aldara treatment. Statistical significance displayed for ΔCT values of Aldara-treated compared with untreated samples of the same strain; * P <0.05, ** P <0.01, *** P <0.001 (unpaired Student’s t -test). Full size image Stressed or dying keratinocytes commonly release IL-1α, a cytokine that stimulates production of keratinocyte mitogens by stromal cells [28] , [29] . To determine a possible role of such paracrine-acting growth factors in the hyperproliferation induced by Aldara treatment, we demonstrated upregulation of IL-1α mRNA levels 24 h after one topical Aldara treatment ( Fig. 2d ). We then performed quantitative real-time PCR (qPCR) analysis to determine the expression of the keratinocyte mitogens Csf2 (granulocyte-macrophage colony-stimulating factor), Csf3 (granulocyte colony-stimulating factor, G-CSF), Hgf (hepatocyte growth factor), Fgf7 (fibroblast growth factor 7) and Tgfα (transforming growth factor α) 24 h after one topical Aldara treatment. We observed a moderate upregulation of the transcripts of Gm-csf and Tgfα and a drastic upregulation of G-csf mRNA levels ( Fig. 2c ). We then confirmed G-csf upregulation also for TLR7-ko, WT129 and A129 mice 24 h after one Aldara application ( Fig. 2e ). To exclude that the effect of Aldara is due to signalling via another TLR, we performed qPCR analysis in MyD88-ko mice. Although we did not see a significant increase in IL-1α expression after Aldara treatment, which maybe due to the described impairments of IL-1α signalling in these mice [30] , G-csf was prominently upregulated in MyD88-ko mice 24 h after one Aldara application ( Supplementary Fig. S6 ). Aldara induces neutrophil infiltration Concomitant with the appearance of apoptotic keratinocytes, we detected neutrophils in close vicinity to apoptotic areas underneath the epidermis 12 h after one Aldara application, which subsequently migrated through the epidermis ( Fig. 3a ). In contrast, the untreated control skin was completely devoid of neutrophils. We observed large neutrophil-filled abscess-like structures at 24 h after one topical Aldara treatment in all mouse strains, similar to the abscesses that are common in psoriatic skin [31] , [32] . The average size of the abscesses was independent of type I IFN and TLR7 signalling ( Fig. 3a ; Supplementary Fig. S7b ). After 1 week of Aldara application, neutrophils were absent from the follicular epidermis, but still sparsely infiltrated the dermis of all mouse strains and were part of the parakeratotic crust ( Fig. 3a ; Supplementary Fig. S7a ). To explain the pronounced recruitment of neutrophils into Aldara-treated epidermis, we assessed expression of the genes encoding S100A8/A9. These are calcium-binding proteins that are expressed by and released from stressed keratinocytes and induce neutrophil migration [33] . The mRNA levels for both proteins were strongly upregulated in Aldara-treated skin 24 h after a single Aldara application ( Fig. 3c ). In addition, we found that expression of neutrophil-attracting chemokine Cxcl1 [34] was strongly upregulated 24 h after Aldara treatment ( Fig. 3e ). The strong infiltration of neutrophils that we observed after Aldara treatment fits with the fact that all inflammasome-related diseases, as well as conditions with an involvement of IL-1, are characterized by an influx of neutrophils. Recently, expression of the cytokine IL-17A was shown to be important for keratinocyte hyperproliferation in Aldara-treated mice, especially after 2 days of Aldara treatment [22] . Furthermore, a recent publication reported that dermal γδ-T cells, expressing the transcription factor RORγt, are a major source of innate IL-17A [8] . We confirmed a strong upregulation of this cytokine already 24 h after one Aldara application ( Fig. 3f ). IL-23 has recently been identified as a crucial mediator of Aldara- and psoriasis-associated epidermal hyperplasia and inflammation [8] , but the initial trigger for IL-23 production in the skin has not been identified. We observed a strong TLR7-independent upregulation of IL-23 24 h after one topical Aldara treatment ( Fig. 3g ), however, IL-23 was not upregulated in Aldara-treated MyD88-ko mice ( Supplementary Fig. S6 ), suggesting MyD88 signalling via IL-1 or another TLR as crucial in the Aldara-mediated induction of IL-23. Aldara-induced IL-17 seems not crucial for the phenotype observed after 24 h, because RORc-ko mice, which lack the transcription factor RORγt and are therefore impaired in IL-17 and IL-22 production [24] , [35] , [36] , displayed acanthosis, epidermal hyperproliferation and scaling to a similar extent as in C57BL/6 controls ( Supplementary Fig. S8 ). However, psoriasis-like lesions evolve only after a number of days following consecutive Aldara treatment, and the loss of RORc halts lesion development beyond the initial signs of inflammation observed after 24 h of treatment [24] . Aldara, but not IMQ, activates inflammasomes in keratinocytes We demonstrated that Aldara treatment resulted in the upregulation of IL-1α transcripts. We next investigated whether other members of the IL-1 family such as IL-1β and IL-18 (ref. 37 ) are produced upon treatment with Aldara. It was shown that IMQ activates the inflammasome in murine peritoneal macrophages, [38] but such evidence is lacking for keratinocytes. Exposure of primary human keratinocytes to Aldara in vitro induced the release of cleaved caspase-1 (caspase-1 CARD domain), mature IL-1β (IL-1β p17) and IL-18 (IL-18 p17) into the cell-culture supernatant ( Fig. 4a ). Using a pan-caspase inhibitor (VAD) or caspase-1 inhibitor (YVAD), we showed that Aldara-induced IL-1β maturation was caspase-1 dependent ( Fig. 4c ). IL-1β maturation was abrogated after small interfering RNA (siRNA)-mediated knockdown of NLRP-1 and ASC but not of NLRP3 expression ( Fig. 4d ), suggesting that Aldara activates the NLRP1 inflammasome. It was recently shown that IMQ itself induces apoptosis in a TLR7-independent fashion [7] , [19] , but there is no evidence that the Aldara vehicle can act on keratinocytes directly. We thus investigated whether IMQ or another component in the Aldara vehicle cream mediates inflammasome activation. As a control, we used a cream that is commonly used as a basis for topically applied medications (softcream). Incubation of keratinocytes with IMQ or softcream did not lead to any of the above-mentioned effects, but incubation of keratinocytes with Aldara vehicle cream mimicked the effects of Aldara ( Fig. 4f ). To exclude the possibility that IMQ had no effect because it was not able to enter the cells, we used lipofectamine2000 to bring IMQ or Aldara directly into keratinocytes. Again, Aldara, but not IMQ, induced secretion of IL-1β by primary human keratinocytes. 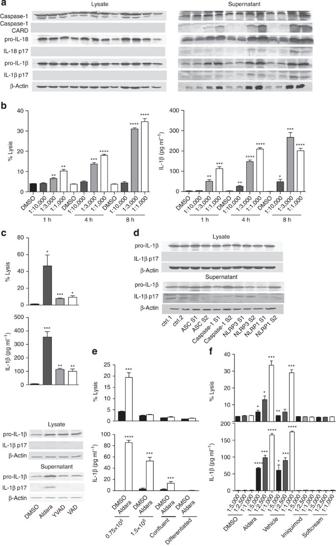Figure 4: Aldara, but not IMQ, activates the inflammasome in human primary keratinocytes. (a) Keratinocytes were treated with different concentrations of Aldara for certain time periods. Whole-cell lysate (left) as well as acetone-precipitated supernatants (right) were resolved by SDS–PAGE. The resulting western blots were probed with the antibodies indicated on the left-hand side. The vehicle DMSO served as negative control. (b) The relative efficiency of cell lysis by the indicated concentrations of Aldara and DMSO 1:1,000 inawas assessed by lactate dehydrogenase (LDH) assays (left) and the amount of released IL-1β inbwas measured by ELISA (right). (c) Thirty minutes before Aldara treatment (1:1,000, 4 h), keratinocytes were pretreated with a pan-caspase inhibitor (VAD, 20 μM) or a caspase-1 inhibitor (YVAD, 50 μM). The efficiency of cell lysis was assessed with LDH assays (top panel), and mature IL-1β release was measured with ELISA (middle panel). Cell lysate and acetone-precipitated supernatants were resolved by SDS–PAGE, and the western blots were probed with the antibodies indicated on the left-hand side (bottom panel). (d) Keratinocytes were transfected with scrambled siRNA (ctrl. 1), with siRNA directed against Caspase-5 (ctrl. 2) or with siRNA directed against ASC, caspase-1, NLRP3 and NLRP1 two days before Aldara treatment (1:3,000, 4 h). Secretion of mature IL-1β into the supernatant was assessed by western blotting using antibodies against pro- IL-1β and IL-1β p17. Probing with an antibody recognizing β-actin served as loading control. (e) Keratinocytes were either seeded at the indicated densities per well into a six-well plate or had been transferred into KBM-2 medium for differentiation 5 days before Aldara treatment (1:3,000, 4 h). The efficiency of cell lysis was assessed with LDH assays (top), and mature IL-1β release was measured with ELISA (bottom). (f) Cells were treated either with DMSO, Aldara, vehicle, IMQ or softcream for 4 h at the indicated concentrations. The efficiency of cell lysis was assessed with LDH assays (top), and mature IL-1β release was measured with ELISA (bottom). Error bars indicate s.d.; *P<0.05, **P<0.01 and ***P<0.001, ****P<0.0001 (unpaired Student’st-test). Figure 4: Aldara, but not IMQ, activates the inflammasome in human primary keratinocytes. ( a ) Keratinocytes were treated with different concentrations of Aldara for certain time periods. Whole-cell lysate (left) as well as acetone-precipitated supernatants (right) were resolved by SDS–PAGE. The resulting western blots were probed with the antibodies indicated on the left-hand side. The vehicle DMSO served as negative control. ( b ) The relative efficiency of cell lysis by the indicated concentrations of Aldara and DMSO 1:1,000 in a was assessed by lactate dehydrogenase (LDH) assays (left) and the amount of released IL-1β in b was measured by ELISA (right). ( c ) Thirty minutes before Aldara treatment (1:1,000, 4 h), keratinocytes were pretreated with a pan-caspase inhibitor (VAD, 20 μM) or a caspase-1 inhibitor (YVAD, 50 μM). The efficiency of cell lysis was assessed with LDH assays (top panel), and mature IL-1β release was measured with ELISA (middle panel). Cell lysate and acetone-precipitated supernatants were resolved by SDS–PAGE, and the western blots were probed with the antibodies indicated on the left-hand side (bottom panel). ( d ) Keratinocytes were transfected with scrambled siRNA (ctrl. 1), with siRNA directed against Caspase-5 (ctrl. 2) or with siRNA directed against ASC, caspase-1, NLRP3 and NLRP1 two days before Aldara treatment (1:3,000, 4 h). Secretion of mature IL-1β into the supernatant was assessed by western blotting using antibodies against pro- IL-1β and IL-1β p17. Probing with an antibody recognizing β-actin served as loading control. ( e ) Keratinocytes were either seeded at the indicated densities per well into a six-well plate or had been transferred into KBM-2 medium for differentiation 5 days before Aldara treatment (1:3,000, 4 h). The efficiency of cell lysis was assessed with LDH assays (top), and mature IL-1β release was measured with ELISA (bottom). ( f ) Cells were treated either with DMSO, Aldara, vehicle, IMQ or softcream for 4 h at the indicated concentrations. The efficiency of cell lysis was assessed with LDH assays (top), and mature IL-1β release was measured with ELISA (bottom). Error bars indicate s.d. ; * P <0.05, ** P <0.01 and *** P <0.001, **** P <0.0001 (unpaired Student’s t -test). Full size image Because murine keratinocytes do not express detectable amounts of pro-IL-1β, IL-18 is the only cytokine in murine skin that requires maturation via the inflammasome to be biologically active [39] . To investigate whether IL-18 contributes to epidermal hyperproliferation, we treated IL-18R-ko mice with Aldara and assessed epidermal thickness. After 1 week of Aldara treatment, we observed that the increase in epidermal thickness was more pronounced in IL-18R-ko mice than in Aldara-treated C57BL/6 controls (increase after 7 days of Aldara-treated IL-18R-ko mice compared with untreated mice: 479% and increase after 7 days of Aldara-treated C57BL/6 compared with untreated mice: 325%, P =0.2). This finding indicates that Aldara also has an impact on the murine inflammasome in vivo. Furthermore, it implicates an attenuating effect of IL-18 on the inflammatory response to Aldara in vivo and fits the recent observations that IL-18 protects against colitis and colitis-associated cancer in mice [40] . Besides activation of the inflammasome, Aldara caused lysis of human keratinocytes in a time- and dose-dependent manner starting 1 h after treatment of the cells ( Fig. 4a ). Keratinocyte cell death was reduced in the presence of pan-caspase or caspase-1 inhibitors ( Fig. 4c ), which provides an explanation for the recently reported TLR7-independent death of keratinocytes [7] . Caspase-1-dependent lysis of keratinocytes is called ‘pyroptosis’, a mechanism that is distinct from apoptosis and independent of apoptosis-related caspases [41] . Aldara-induced inflammasome activation and death of keratinocytes were more pronounced in subconfluent (proliferating) keratinocyte cultures, and both effects were abolished in differentiated keratinocytes ( Fig. 4e ). Taken together, by inducing rapid keratinocyte death, Aldara results in the release of IL-1α and the downstream effects described above. In addition, Aldara activates the inflammasome, which results in the release of pro-IL-1α and production of IL-1β, IL-18 and maybe also other members of this family such as IL-36. Full local response requires Aldara vehicle plus IMQ Only Aldara and vehicle cream, but not IMQ, induced activation of the inflammasome and cell lysis in human keratinocytes in vitro , suggesting that components of the vehicle are responsible for these early effects. To explore this further in vivo , we treated WT129 mice with Aldara, vehicle cream, IMQ solubilized in softcream or IMQ solubilized in vehicle and performed qPCR for selected cytokines 24 h later. Both, vehicle alone (that is, no IMQ) and IMQ/softcream (that is, no vehicle components), induced comparable upregulation of the transcripts for IL-1α, G-CSF, S100A8, S100A9, IL-17A and IL-23 ( Fig. 5a–f ), although less pronounced compared with Aldara or IMQ/vehicle (that is, vehicle components plus IMQ). Along the same lines, Aldara, IMQ/softcream and vehicle induced parakeratosis, whereas softcream did not, although only Aldara resulted in significant skin thickening ( Supplementary Fig. S9a ). However, vehicle alone did induce a significant increase in TUNEL + keratinocytes ( Supplementary Fig. S9b ). 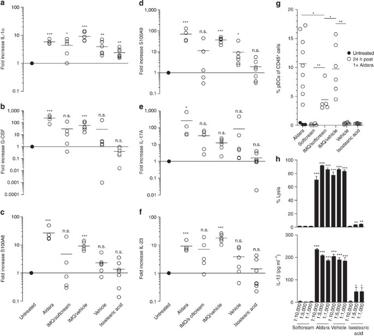Figure 5: IMQ and vehicle alone induce cytokine production in WT129 skin. mRNA levels ofIl-1α(a),G-csf(b),S100A8(c),S100A9(d) andIl-17A(e) andIl-23(f) in the skin of WT129 mice assessed by qPCR 24 h after one topical treatment. Statistical significance displayed for ΔCT values of treated compared with untreated samples. (g) pDC mobilization in the blood of WT129 mice 24 h after one topical treatment, lyophilized IMQ solubilized in softcream (IMQ/softcream), IMQ solubilized in vehicle (IMQ/vehicle), vehicle cream, softcream or isostearic acid in softcream (25% w/w). (h) Human primary keratinocytes were treated at the indicated concentrations with DMSO-solubilized softcream, Aldara, vehicle or isostearic acid for 6 h. The relative efficiency of cell lysis was assessed by LDH assays (top), and the amount of released IL-1β was measured by ELISA (bottom). Statistical significance displayed for all samples treated with Aldara, vehicle or isostearic acid in softcream compared with the corresponding concentration of softcream alone; error bars indicate s.d.; *P<0.05, **P<0.01, ***P<0.001, ****P<0.0001, n.s. (P>0.5 not significant) unpaired Student’st-test. Figure 5: IMQ and vehicle alone induce cytokine production in WT129 skin. mRNA levels of Il-1α ( a ), G-csf ( b ), S100A8 ( c ), S100A9 ( d ) and Il-17A ( e ) and Il-23 ( f ) in the skin of WT129 mice assessed by qPCR 24 h after one topical treatment. Statistical significance displayed for ΔCT values of treated compared with untreated samples. ( g ) pDC mobilization in the blood of WT129 mice 24 h after one topical treatment, lyophilized IMQ solubilized in softcream (IMQ/softcream), IMQ solubilized in vehicle (IMQ/vehicle), vehicle cream, softcream or isostearic acid in softcream (25% w/w). ( h ) Human primary keratinocytes were treated at the indicated concentrations with DMSO-solubilized softcream, Aldara, vehicle or isostearic acid for 6 h. The relative efficiency of cell lysis was assessed by LDH assays (top), and the amount of released IL-1β was measured by ELISA (bottom). Statistical significance displayed for all samples treated with Aldara, vehicle or isostearic acid in softcream compared with the corresponding concentration of softcream alone; error bars indicate s.d. ; * P <0.05, ** P <0.01, *** P <0.001, **** P <0.0001, n.s. ( P >0.5 not significant) unpaired Student’s t -test. Full size image In contrast to local effects on the skin, which appeared to be largely independent of IMQ and TLR7, pDC mobilization required the presence of IMQ ( Fig. 5g ), excluding the presence of an unknown TLR7 ligand in the vehicle. The fact that pDC mobilization was less pronounced after treatment with IMQ/softcream maybe explained by diminished bioavailability of IMQ when applied in softcream. Our data suggest that a vehicle component is sufficient to induce keratinocyte death (pyroptosis) and concomitant IL-1α release followed by some downstream effects, but involvement of TLR7 + cells is required for the full local response. On the other hand, signalling through TLR7 + cells only, which implies no involvement of keratinocytes, may produce an attenuated inflammatory phenotype because the contribution of dying keratinocytes and immediate IL-1α is lacking. According to the US patent 7696159, isostearic acid (25% w/w) is the second most abundant component in Aldara after water. It was shown recently that fatty acids can activate inflammasomes [42] , [43] , thus we investigated whether isostearic acid contributes to the effect of vehicle on keratinocytes. We treated primary human keratinocytes with isostearic acid (25% w/w in softcream) in vitro and observed lysis of keratinocytes and inflammasome activation as illustrated by IL-1β release ( Fig. 5h ). Induction of keratinocyte lysis was abrogated by siRNA-mediated knockdown of caspase-1 ( Supplementary Fig. S10 ). Subsequently, we topically treated WT129 mice with isostearic acid (25% w/w in softcream) and determined the mRNA levels of IL-1α, G-CSF, IL-17A, IL-23, S100A8 and S100A9 in the treated skin using qRT–PCR. Although only statistically significant for IL-1α ( P =0.0035), isostearic acid induced upregulation of some additional transcripts ( Fig. 5a–f ), suggesting a contribution of the vehicle component, isostearic acid, to the immediate skin inflammation induced by Aldara. Based on the level of transcripts, isostearic acid may contribute to inflammasome activation and pyroptosis in keratinocytes, with concomitant secretion and release of IL-1α, whereas some of the downstream pathways are influenced by other vehicle components and/or IMQ. Aldara induces keratinocyte proliferation in human NMSC Because induction of proliferation is an unanticipated effect of an anti-cancer treatment, we investigated whether Aldara-induced proliferation of keratinocytes also occurs in NMSC patients and patients with precursor lesions. We therefore stained biopsies that were taken before and after Aldara treatment from six BCC and four AK patients for Ki67. Aldara treatment increased proliferation of malignant and pre-malignant epidermal keratinocytes in all cases ( Fig. 6a ). In several cases, increased Ki67 staining was even observed in nonmalignant peritumoral epidermis ( Fig. 6f ). Furthermore, we observed substantial infiltration of cells expressing myeloperoxidase (MPO), a common human neutrophil marker. Although almost absent in untreated skin from AK and BCC patients, MPO + cells represented between 30 and 90% of the overall strongly increased immune cell infiltration in both types of lesions ( Fig. 6c ) after Aldara treatment. In addition, BCC and AK commonly displayed a parakeratotic crust filled with neutrophils, which strongly resembled the murine Aldara-induced skin inflammation ( Figs 3b and 6c ). 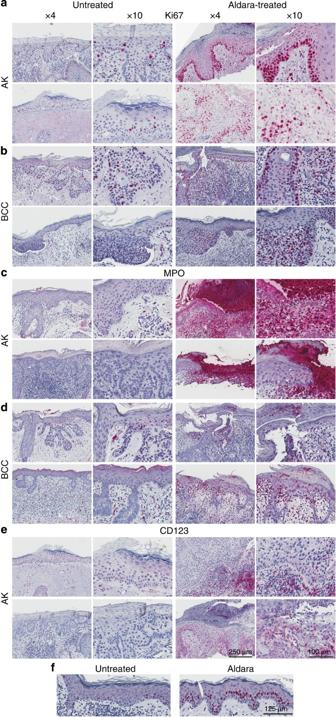Figure 6: Hyperproliferation and infiltration of neutrophils and pDC in Aldara-treated human BCC and AK. Ki67 (a), MPO (c) and CD123 (e) staining of two representative AK lesions before and after 2 weeks of Aldara therapy. Ki67 (b) and MPO (d) staining of two representative BCC lesions and Ki67 (f) staining of peritumoral epidermis before and 5 days after Aldara therapy. For clarity, imagesa–dwere acquired in two different magnifications (× 4 and × 10). Scale bar, 250 μm (for × 4 magnification) and 100 μm (for × 10 magnification). Scale bar, 125 μm (f). Figure 6: Hyperproliferation and infiltration of neutrophils and pDC in Aldara-treated human BCC and AK. Ki67 ( a ), MPO ( c ) and CD123 ( e ) staining of two representative AK lesions before and after 2 weeks of Aldara therapy. Ki67 ( b ) and MPO ( d ) staining of two representative BCC lesions and Ki67 ( f ) staining of peritumoral epidermis before and 5 days after Aldara therapy. For clarity, images a – d were acquired in two different magnifications (× 4 and × 10). Scale bar, 250 μm (for × 4 magnification) and 100 μm (for × 10 magnification). Scale bar, 125 μm ( f ). Full size image pDCs have been reported as the most prominent cell type infiltrating BCC following Aldara treatment [6] and as crucial for Aldara-dependent anti-tumour effects in murine melanoma [7] . To investigate whether this is also the case in human AK, we stained four AK sections with CD123, a marker for human pDCs. Although pDCs were almost absent in AK before treatment, they became a substantial part of the peritumoral infiltrate following Aldara treatment, but were not part of the parakeratotic crust ( Fig. 6e ) and were outnumbered by neutrophils in all samples analysed. Aldara induces epidermal hyperplasia [22] , suggesting a direct impact on TLR7-negative normal and transformed keratinocytes. Indeed, we found that Aldara induces a plethora of TLR7- and even IMQ-independent inflammatory events in healthy and malignant human and murine skin. Based on our data, we propose that one of the first responses to topical Aldara application is the induction of keratinocyte death, part of which presumably depends on NLRP1 inflammasome activation (pyroptosis) and concomitant release of IL-1α. Keratinocytes express large amounts of pro-IL-1α, which is biologically active without further processing. It is released upon cell lysis and can be secreted after inflammasome activation [39] , [44] . IL-1 can act in an autocrine manner, and its release by dying keratinocytes can stimulate further IL-1 production [39] . In addition, it induces production of major keratinocyte mitogens by fibroblasts [45] , [46] . We found that Aldara also activated the NLRP-1 inflammasome in (human) keratinocytes resulting in caspase-1-dependent production of biologically active IL-1β. In addition, Aldara induces expression of G-CSF production by fibroblasts and the induction of S100A8/A9 [28] , [29] and IL-23 production by dermal myeloid cells, which in turn induces IL-17 secretion by dermal γδ-T cells [8] . IL-17 and G-CSF have an impact on keratinocytes resulting in their proliferation, whereas S100A8/A9 and CXCL1 are strong chemoattractants for neutrophils. The observed local inflammatory changes and epidermal hyperplasia are reminiscent of psoriasis [8] , [23] , [32] , [47] . Hyperproliferation and psoriatic plaques induced by Aldara have primarily been ascribed to cytokines, such as IL-17 (refs 8 , 22 ) and IL-22 (ref. 23 ). By utilizing RORc-ko mice, however, we found that IL-17 does not seem to be required for the early keratinocyte response to Aldara. Nevertheless, inflammation and acanthosis were reduced in RORc-ko mice after 7 days of daily Aldara treatment [24] , suggesting a role for IL-17 in propagation rather than in initiation of the inflammation. Strikingly, we found that vehicle, but not IMQ, induced keratinocyte lysis, inflammasome activation and IL-1 release in keratinocytes in vitro within 4 h of treatment. This stands in contrast to recent data, suggesting that IMQ alone can activate the inflammasome in macrophages and induce apoptosis in murine keratinocytes after a 40-h treatment [7] , [38] . As this study focuses on the early Aldara-mediated events in keratinocytes, our data do not exclude the possibility that IMQ may activate the inflammasome in different cell types or induce apoptosis in human keratinocytes at later time points. We identified isostearic acid, which makes up to 25% of the vehicle and is the most abundant component after water, as a component with biological activity in the context of skin inflammation. For example, isostearic acid mimicked the effect of vehicle in primary human keratinocytes in vitro (apoptosis, inflammasome activation and IL-1 release) and increased expression of cytokines in vivo , suggesting that isostearic acid is one of the active components of Aldara. This fits with observations that describe the direct activation of inflammasomes by fatty acids [42] , [43] . Despite the induction of keratinocyte apoptosis and downstream pathways in vitro , the vehicle or IMQ in softcream failed to induce the full skin phenotype in vivo , indicating that IMQ and vehicle components execute additive or synergistic actions. This newly discovered IMQ-independent activity of Aldara might explain the therapeutic efficacy of the placebo, which was observed in most clinical trials that included a placebo-control group [1] , [2] , [48] . The fact that the clinical response of Aldara-treated patients was always greater than that of the placebo-treated patients suggests that the IMQ-dependent and -independent pathway must act in concert for optimal efficacy. Collectively, our data suggest that Aldara induces cell death and inflammasome activation in keratinocytes. Caspase-1-dependent cell death (pyroptosis) results in the release of IL-1α. Inflammasome activation results in the release of pro-IL-1α and the maturation of pro-IL-1β to the biologically active IL-1β. Furthermore, Aldara induces G-CSF (fibroblasts) and IL-23 (dermal myeloid cells). IL-1 and G-CSF induce keratinocyte proliferation. IL-23 induces proliferation of resident dermal γδ T cells as well as production of IL-17 by the latter, and may also recruit other IL-17-producing cells. Moreover Aldara induces S100A8/A9 and CXCL1 release, which are strong chemoattractants for neutrophils as is IL-1 (graphic summary in Fig. 7 ). 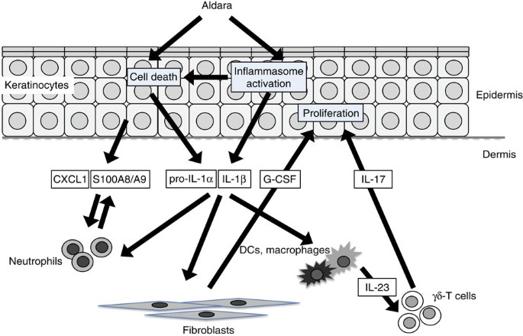Figure 7: Schematic representation of novel TLR7-independent Aldara-induced events in the skin. Aldara induces cell death and inflammasome activation in keratinocytes. Caspase-1-dependent cell death (pyroptosis) results in the release of IL-1α. Inflammasome activation results in the release of pro-IL-1α and the maturation of pro-IL-1β to the biologically active IL-1β. Furthermore, Aldara induces G-CSF (fibroblasts) and IL-23 (dermal myeloid cells). IL-1 and G-CSF induce keratinocyte proliferation. IL-23 induces proliferation of resident dermal γδ T cells as well as production of IL-17 by the latter and may also recruit other IL-17-producing cells. Moreover, Aldara induces S100A8/A9 and CXCL1 release, which are strong chemoattractants for neutrophils as is IL-1. Figure 7: Schematic representation of novel TLR7-independent Aldara-induced events in the skin. Aldara induces cell death and inflammasome activation in keratinocytes. Caspase-1-dependent cell death (pyroptosis) results in the release of IL-1α. Inflammasome activation results in the release of pro-IL-1α and the maturation of pro-IL-1β to the biologically active IL-1β. Furthermore, Aldara induces G-CSF (fibroblasts) and IL-23 (dermal myeloid cells). IL-1 and G-CSF induce keratinocyte proliferation. IL-23 induces proliferation of resident dermal γδ T cells as well as production of IL-17 by the latter and may also recruit other IL-17-producing cells. Moreover, Aldara induces S100A8/A9 and CXCL1 release, which are strong chemoattractants for neutrophils as is IL-1. Full size image In conclusion, we uncovered unexpected effects of Aldara on human and mouse keratinocytes, which are independent of TLR7 and even independent of the major active compound IMQ. With respect to these new findings, it will be important to investigate the relevance of the TLR7-dependent and -independent pathways for the therapeutic effect of Aldara. Mice C57BL/6 (C57BL/6JOlaHsd), WT129 (129S6/SvEvTac), type I IFN receptor knockout (ko) (A129, 129Sv/Ev-IFNabR<tm1Agt>) [49] , TLR7-ko (B6-TLR7<tm1aki>) [50] and MyD88-ko (B6.129P2-Myd88<tm1aki>) [30] mice were obtained from the Institute of Laboratory Animal Science (University of Zurich, Zurich, Switzerland), Harlan Laboratories (Indianapolis, IN, USA) or Taconic (Germantown, NJ, USA); IL-18R-ko (B6-IL18R<tm1aki>) [51] and RORc-ko mice (B6.129P2(Cg)-Rorc<tm2Litt>) [52] were provided by Burkhard Becher (University of Zurich, Zurich, Switzerland). All mice were bred and maintained under specific pathogen-free conditions. Experiments were performed with female mice of 6–8 weeks in accordance with the Swiss federal and cantonal laws on animal protection. In vivo Aldara application Aldara (5% IMQ cream, source throughout the entire study: Meda Pharma, Wangen-Brüttisellen, Switzerland), softcream (Kantonsapotheke, Zurich, Switzerland; ingredients (w/w): 32.5% paraffin, 22.7% white petrolatum, 3.2% glycerol monostearat 40–50, 2.1% sorbitanmonostearat, 4.4% polyoxyl ethylene glycol(30)-stearat, 0.1% citric acid monohydrate, 21% H 2 O, 5% urea, 8.5% glycerin 85%, 0.5% phenotexol), 5% IMQ (lyophilized; Biovision, Mountain View, CA, USA) in softcream, 5% IMQ in vehicle (3M, St. Paul, MN, USA; previous owner of ‘Aldara’, pharmaceutical division Europe sold to Meda Pharma in 2006), and vehicle alone or 25% isostearic acid in softcream were applied topically for 24 h (one application) or 7 days (four applications, last application 24 h before collection of skin) on the shaved back skin of mice, and the mice were carefully creamed to allow penetration of the compounds. Patient samples All patients enroled in the study were treated at the Department of Dermatology, University Hospital of Zurich. The cantonal ethics committee (EK no. 647) approved this study, and all patients signed a declaration of informed consent. Biopsies were obtained from eight BCC patients before and 1 week after start of Aldara treatment (5 × per week), and from four AK patients before and 2 weeks after start of Aldara treatment (3 × per week). Biopsies were surgically excised and stored in formalin. RNA isolation, reverse transcription PCR and qRT–PCR Samples were stored in RNA later, and total RNA extraction was performed with TRIzol (Invitrogen, Carlsbad, CA, USA). RNA was subjected to DNase I digestion (Invitrogen), and total RNA concentration and purity were evaluated using the NanoDrop ND-1000 spectrophotometer (Thermo Scientific, Wilmington, DE, USA). RNA (500 ng) was reverse transcribed using the High-Capacity cDNA Reverse Transcription Kit (Applied Biosciences, Carlsbad, CA, USA). The screen for keratinocyte mitogens was performed with the SYBR green system. A volume of 0.5 μl of cDNA (produced as described above) was used for quantitative RT–PCR, using a Light Cycler 480 (Roche, Basel, Switzerland), 10 nM primers and 2x Light Cycler 480 SYBR green I mix (Roche) in a 25-μl reaction volume. Gapdh primers were used for normalization. The following primers were used: Gapdh: 5′-TCGTGGATCTGACGTGCCGCCTG-3′, 3′-CACCACCCTGTTGCTGTAGCCGTAT-5′; Csf2: 5′-TCATTTTTGGCCTGGTTTTT-3′, 3′-TATTCGAGCAGGGTCTACGG-5′; Csf3: 5′-TGCACTATGGTCAGGACGAG-3′, 3′-GGGGTGACACAGCTTGTAGG-5′; Hgf: 5′-TTTGCTTTAGGGATCAGTCTG-3′, 3′-GGCCTTGCAAGTGAAC-5′; Fgf7: 5′-CAAACGGCTACGAGTGTGAA-3′, 3′-CCTTTGATTGCCACAATTCC-5′; Tnfa: 5′-GACCCTCACACTCAGATCATCTTCT-3′, 3′-CCACTTGGTGGTTTGCTACGA-5′. All other qRT–PCRs were performed with the TaqMan system (Applied Biosystems, Carlsbad, CA, USA). A volume of 1 μl of cDNA (produced as described above) was used in a 10-μl reaction of TaqMan Master mix and TaqMan assay (Applied Biosystems). Expression was normalized to Gapdh. The following TaqMan assays were used: Gapdh (TaqMan assay: Mm99999915_g1), S100a8 (Mm00496696_g1), S100a9 (Mm00656925_m1), Il1α (Mm00439620_m1), IL-17A (Mm00439618_m1), Il-18 (Mm00434225_m1), Il-23 (Mm00518984_m1), Csf3 (Mm00438334_m1) and CXCL1 (Mm04207460_m1). Immunohistochemistry and immunofluorescence Processing and staining of human tissues: paraffin-embedded tissue sections were stained with mouse anti-human monoclonal antibody against Ki67, polyclonal rabbit anti-human MPO (Dako, Baar, Switzerland) and mouse anti-human monoclonal antibody against CD123 (BD Biosciences Pharmingen, Basel, Switzerland). Sections were counterstained with hematoxylin, dehydrated and mounted. All stainings were performed on a Dako IH with the Dako REAL Detection System (Dako). Sections were counterstained with hematoxylin, dehydrated, mounted, scanned with ScanScope CS (Aperio Technologies, Vista, CA, USA) and analysed with ImageScope version 10.2.1 (Aperio). Processing and staining of mouse tissues: for immunofluorescence, formalin-fixed, paraffin-embedded sections were stained with rabbit anti-mouse monoclonal antibodies against K10, K14, K6, K16, loricrin (Covance, Berkeley, CA, USA) and goat anti-rabbit Cy3 (Jackson ImmunoResearch, West Grove, PA, USA). For immunohistochemistry, HOPE-fixed and low-melting paraffin (DCS, Hamburg, Germany)-embedded tissues were stained with the monoclonal antibodies rabbit anti-mouse Ki67 (Thermo Scientific), rat anti-mouse Ly6G, rat anti-mouse CD45, hamster anti-mouse gdTCR (all from BD Biosciences Pharmingen), hamster anti-mouse CD11c (AbD Serotec, Dusseldorf, Germany), rabbit anti-mouse CD3 (Thermo Scientific) and the polyclonal antibody rabbit anti-mouse-cleaved caspase 3 (Cell Signaling, Danvers, MA, USA). Secondary antibodies: rabbit anti-hamster (Novus Biologicals, Cambridge, UK) and rabbit anti-rat (Jackson ImmunoResearch). Detection was performed with Refine-AP-Kit on BenchMark (Leica, Wetzlar, Germany), using Leica reagents for the entire procedure. TUNEL assays were performed on 3.0 μm paraffin sections of tissue that had been fixed in 4% formalin in PBS using DIG-11-dUTP (Roche), TdT-Buffer and TdT Enzyme (Promega, Madison, WI, USA). Detection was performed with biotinylated mouse anti-digoxigenin followed by Leica Intense-R-HRP Kit on BenchMark (Leica). Sections were counterstained with hematoxylin, dehydrated and mounted. All immunohistochemistry of mouse tissues was performed by Sophistolab, Eglisau, Switzerland. Immunohistochemical stainings were photographed using a Zeiss Axioskop 2 microscope with an Axiocam HRc camera and the Axiovision 4.2 software. Immunofluorescence stainings were photographed using a Zeiss Axio Imager.A1 microscope with an Axiocam MRm camera and the Axiovision 4.6 software (all from Zeiss, Oberkochen, Germany). Adobe Photoshop CS5 version 12.0 (Adobe Systems, Inc., San Jose, CA, USA) was used for image analysis. Electron microscopy Mouse skin samples were excised and immediately transferred to 4% paraformaldehyde in PBS, fixed overnight, rinsed and stored in PBS. Before embedding, samples were treated with 2% OsO4 for 2 h. After washing, they were stained in 1% uranyl acetate, dehydrated through a series of graded ethanols and embedded in Araldite resin. Ultra-thin sections (30–60 nm) were processed with a diamond knife and placed on copper grids. Transmission electron microscopy was performed using a EM 902A electron microscope (Zeiss) with Megaview III digital image acquisition system and analysed with iTEM software, version 5.0. Morphometric analyses and histological quantifications Epidermal thickness was determined by measuring the interfollicular epidermal area including or excluding parakeratotic areas and corresponding length on hematoxylin and eosin-stained longitudinal paraffin sections (6 μm) from mouse back skin. Quantification of the size of abscesses and TUNEL + cells were performed on TUNEL-stained paraffin sections (6 μm) from mouse back skin. Analyses were performed using the Openlab 3.1.5 software (PerkinElmer, Waltham, MA). Flow cytometry Blood or bone marrow was collected in FACS buffer (PBS+2% FCS+40 mM EDTA+0.05% NaN 3 ) and stained with the following antibodies: CD3 FITC, CD19 FITC, Dx5 FITC, c-kit FITC, Sca-1 PE, PDCA-1 PE, CD45.2 PerCp, SiglecH pacific blue, MHC-II pacific blue and CD11c APC (BioLegend, San Diego, CA, USA). Samples were measured with a CyAn ADP9 (Beckman Coulter, Brea, CA, USA) and analysed using FlowJo Analysis Software (Tree Star Inc, Ashland, OR, USA). Cell culture and treatment of primary human keratinocytes Human foreskin keratinocytes were isolated and cultured in K-SFM with epidermal growth factor (EGF) and bovine pituitary extract (BPE) (Invitrogen, Basel, Switzerland) as described [44] , [53] . Briefly, keratinocytes were seeded after the third passage at a density of 1.5 × 10 6 per ml or as indicated. The medium was changed the next day and the cells were treated as described. A total of 250 mg Aldara, vehicle, softcream or isostearic acid in softcream (25% w/w) was dissolved in 1.5 ml dimethylsulphoxide (DMSO), 12.5 mg IMQ (Enzo Life Sciences, Lausen, Switzerland) in 1.75 ml DMSO. VAD and YVAD (Enzo Life Sciences) were dissolved in DMSO and used at 20 and 50 μM, respectively. To bring IMQ and Aldara into keratinocytes, 1 μl IMQ/Aldara was dissolved in 100 μl K-SFM (without EGF/BPE) and mixed with 100 μl K-SFM (without EGF/BPE) containing 3 μl Lipofectamine2000. After 20 min, the mixture was added to keratinocytes in a 12-well after medium change. Supernatant and lysate were collected after 16 h. siRNA transfection Transfection of keratinocytes with siRNA has been described. [44] , [53] Briefly, siRNAs (Sigma, Munich, Germany) were dissolved in 200 μl K-SFM without EGF and BPE (final concentration 10 nM), and 1 μl interferin (Polyplus, Illkirch, France) was added. After 10 min, the mixture was added to 1 ml of fresh medium of keratinocytes (with EGF and BPE). Western blotting Western blotting was performed as described. [44] , [53] Briefly, 8–18% polyacrylamide gels were loaded with a lysate or cell supernatant from approximately 3 × 10 4 or 0.9 × 10 5 keratinocytes, respectively. The following antibodies were used for detection: Rabbit anti-caspase-1 (sc-622; Santa Cruz Biotechnology, Santa Cruz, CA), mouse anti-β-actin (A5441; Sigma), mouse anti-IL-1β (MAB201, R&D Systems, Minneapolis, MN), rabbit anti-IL-18 (PM014; MBL, Nagoya, Japan), mouse anti-keratin10 (M700201; Dako), rabbit anti-ASC (ALX-210-905) and mouse anti-NALP1 (ALX-210-904) (both from Enzo Life Sciences). Secondary antibodies were from Promega and development was performed with NBT/BCIP (Promega). ELISA Mouse IFNα was measured with the VeriKine Mouse Interferon-Alpha ELISA Kit (PBL, Piscataway, NJ, USA). Human IL-1β was measured with the DuoSet ELISA (R&D Systems), and lysis was assessed with the lactate dehydrogenase assay (Promega) according to the instructions of the manufacturer. Statistical analysis Statistics were done using the unpaired Student’s two-tailed t- test. Error bars represent s.d. P -values <0.05 were considered significant. How to cite this article: Walter, A. et al . Aldara activates TLR7-independent immune defence. Nat. Commun. 4:1560 doi: 10.1038/ncomms2566 (2013).